A short N-terminal domain of HDAC4 preserves photoreceptors and restores visual function in retinitis pigmentosa Retinitis pigmentosa is a leading cause of inherited blindness, with no effective treatment currently available. Mutations primarily in genes expressed in rod photoreceptors lead to early rod death, followed by a slower phase of cone photoreceptor death. Rd1 mice provide an invaluable animal model to evaluate therapies for the disease. We previously reported that overexpression of histone deacetylase 4 (HDAC4) prolongs rod survival in rd1 mice. Here we report a key role of a short N-terminal domain of HDAC4 in photoreceptor protection. Expression of this domain suppresses multiple cell death pathways in photoreceptor degeneration, and preserves even more rd1 rods than the full-length HDAC4 protein. Expression of a short N-terminal domain of HDAC4 as a transgene in mice carrying the rd1 mutation also prolongs the survival of cone photoreceptors, and partially restores visual function. Our results may facilitate the design of a small protein therapy for some forms of retinitis pigmentosa. Rod and cone photoreceptors of the vertebrate eye are the primary sensory neurons that initiate vision. Many different mutations directly affect these cells, leading to loss of function and degeneration. One such group of diseases, retinitis pigmentosa (RP), is caused by mutations primarily in rod-specific genes [1] . The disease process is initiated in rods, which detect signals in dim light and provide night vision. RP thus first presents as loss of night vision. Unfortunately, cones, which carry out daylight and colour vision, also eventually become dysfunctional in RP patients and die, secondary to rod death. Rd1 mice, one of the most commonly used animal models of RP, carry a mutation in the rod-specific gene PDE6β (phosphodiesterase 6β subunit), which is also mutated in a subset of RP patients [2] , [3] , [4] . The rd1 mutation causes rapid and early rod death, followed by cone death, providing an excellent model for human RP. Several therapeutic strategies have been shown to delay photoreceptor death in rd1 mice, with treatments including neurotrophic factors [5] , calcium channel blockers [6] , antioxidants [7] or anti-apoptosis gene transfer [8] . Histone deacetylase 4 (HDAC4) plays an essential role in supporting the survival of cortical neurons, cerebellar neurons and retinal neurons [9] , [10] , [11] . Altered HDAC4 regulation has been linked to a number of neurodegenerative disorders, such as Parkinson’s disease [12] , [13] , [14] and ataxia [15] , [16] . We previously reported that overexpression of HDAC4 in rd1 mice prolongs rod photoreceptor survival [11] . As HDAC4 is a relatively large protein with a deacetylase domain and multiple other domains that interact with transcription factors and cofactors [17] , [18] , [19] , as well as other HDACs, we conducted a structure–function analysis to determine the essential domain(s) required to promote rod survival. Surprisingly, a short amino terminal domain, devoid of the majority of the defined functional domains of HDAC4, was able to prolong rod survival. This domain is glutamine rich and saved even more rods than full-length HDAC4. The greater rod protection efficiency of the N-terminal domain of HDAC4 at least partly involved greater protein stability. HDAC4 functions in the cytoplasm to suppress multiple pathways involved in photoreceptor death. Rods preserved by HDAC4 in rd1 mice are unlikely to function due to the mutation in PDE6β, an essential gene in rod phototransduction. RP patients maintain functional vision for a long period of time after rod degeneration by relying on the remaining function of cones, which are genetically normal. Therefore, saving cones is key to preserving vision in RP. Significantly, expressing a short N-terminal domain of HDAC4 as a transgene in rd1 mice also prolonged the survival of cones, and as a result, partially restored visual function. A short N-terminal domain of HDAC4 preserves rd1 rods The deacetylase domain of HDAC4 resides in the C-terminal portion of the protein. As a member of Class IIa HDACs, the enzymatic activity of HDAC4 is evolutionarily weak, about 1,000-fold less active than Class I HDACs on standard substrates [20] . In cultured cortical neurons, reduction in HDAC4 expression results in loss of all types of neurons without affecting the survival of astrocytes, and the HDAC4 C-terminal catalytic domain is dispensable for neuroprotection [9] . HDAC4 overexpression also protects cultured cerebellar granule cells from low potassium-induced apoptosis [10] . In order to determine the minimal domain(s) required for rod survival, several deletions of HDAC4 ( Fig. 1a ) were tested in rd1 mice of the FVB strain background. Deletion alleles were constructed in a plasmid using the broadly active CAG promoter and were tested by electroporation in vivo into the subretinal space of rd1 mice at postnatal day 0 (P0). In addition to the HDAC4 plasmid, a CAG-GFP plasmid was included, to mark electroporated cells, along with a Rho-DsRed reporter plasmid that uses the rhodopsin cis-regulatory element to drive expression of DsRed, and thereby mark rod photoreceptors [21] . In rd1 mice, rods die rapidly, with nearly complete rod death by P36 (refs 2 , 4 , 7 , 22 ). The survival of rods was assessed at P50 on retinal flat mounts by examination of Rho-DsRed-positive cells in areas that were well marked by GFP expression. Overexpression of HDAC4 preserved many DsRed-expressing rods, which were also positive for anti-rhodopsin immunoreactivity ( Fig. 1b ). We quantified the overlap between GFP, DsRed and the native marker for rods ( Supplementary Fig. 1 ). About 98.2% Rho-DsRed-positive cells were positive for anti-rhodopsin immunoreactivity, indicating that the Rho-DsRed reporter faithfully labels native rods. And nearly all (99.8%) of Rho-DsRed-positive cells were also positive for GFP, indicating high co-transfection efficiency by in vivo electroporation. The protection effect was not due to the experimental procedure per se , as overexpressing GFP alone did not preserve rods ( Fig. 1b control). Remarkably, overexpression of residues 1–747 of HDAC4, which lacks the deacetylase domain [10] , preserved many more rods than the full-length HDAC4. By contrast, overexpression of residues 612–1,084 of HDAC4 (ref. 17 ) had no protective effect ( Fig. 1c ), indicating that the catalytic domain is dispensable for rod survival through HDAC4 overexpression. 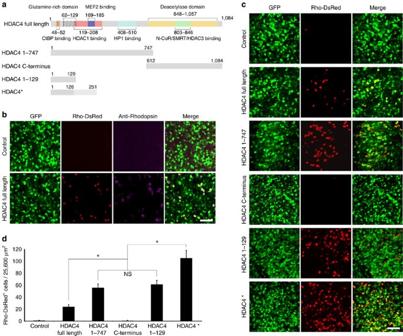Figure 1: Preservation of rod photoreceptors by HDAC4 deletion alleles in rd1 mice. (a) Schematic representation of HDAC4 functional domains and HDAC4 deletion alleles. (b) Co-electroporation of CAG-GFP (transfection marker), CAG-HDAC4 Full Length, and a rhodopsin reporter construct, Rho-DsRed, in the P0 rd1 retinas with assay at P50 for anti-rhodopsin immunoreactivity. Scale bar, 40 μm. (c) Rho-DsRed+rods saved by HDAC4 deletion alleles at P50 in the rd1 retina. Scale bar, 40 μm. (d) Quantification of rod survival by HDAC4 Full Length and HDAC4 deletion alleles. Rho-DsRed-positive cells were scored per 25,600 μm2in transfected areas. *P<0.01. Data are presented as mean±s.d.,n=5–8. Figure 1: Preservation of rod photoreceptors by HDAC4 deletion alleles in rd1 mice. ( a ) Schematic representation of HDAC4 functional domains and HDAC4 deletion alleles. ( b ) Co-electroporation of CAG-GFP (transfection marker), CAG-HDAC4 Full Length, and a rhodopsin reporter construct, Rho-DsRed, in the P0 rd1 retinas with assay at P50 for anti-rhodopsin immunoreactivity. Scale bar, 40 μm. ( c ) Rho-DsRed + rods saved by HDAC4 deletion alleles at P50 in the rd1 retina. Scale bar, 40 μm. ( d ) Quantification of rod survival by HDAC4 Full Length and HDAC4 deletion alleles. Rho-DsRed-positive cells were scored per 25,600 μm 2 in transfected areas. * P <0.01. Data are presented as mean±s.d., n =5–8. Full size image The N-terminal portion of HDAC4 interacts with several proteins that may mediate its pro-survival effect in rd1 rods, including the neuronal survival factor MEF2 (refs 15 , 23 ). Interestingly, a short HDAC4 N-terminal domain incapable of interacting with MEF2, residues 1–129, carries a prominent glutamine-rich region that folds into an α-helix structure [24] . Overexpression of this short N-terminal domain (residues 1–129) of HDAC4 produced a rod protection effect as robust as HDAC4 residues 1–747 ( Fig. 1c ). In addition, we inadvertently made an HDAC4 construct, which we term HDAC4*. This construct exhibited even greater efficiency in saving rd1 rods than the full-length HDAC4 protein or HDAC4 residues 1–129 ( Fig. 1c ). DNA sequencing of HDAC4* revealed a premature stop codon due to the insertion of a repeated sequence ( Supplementary Fig. 2a ). Translation of the HDAC4* sequence predictably produces a protein of 251 residues containing HDAC4 residues 1–126 with an extension of 125 residues translated from the repeated sequence ( Supplementary Fig. 2b ). To verify the protein identity of HDAC4*, we performed a mass spectrometry assay of immunopurified HDAC4* from transfected HEK293T cells with an antibody raised against the N-terminal amino acids 1–19 of HDAC4 ( Supplementary Fig. 2c ). Peptides identified by mass spectrometry confirmed the predicted protein sequence of HDAC4* ( Supplementary Fig. 2d ). Overexpression of the repeated sequence itself, HDAC4* residues 108–251 ( Supplementary Fig. 2e ), did not save rd1 rods ( Supplementary Fig. 2f ). The number of rods preserved by HDAC4 deletion alleles was quantified per 25,600 μm 2 in the electroporated areas labelled by co-electroporated CAG-GFP on retinal flat mounts ( Fig. 1d ). While HDAC4 Full Length saved 24.1±3.6 (mean±s.d., n =5) rods, the number of rods preserved by HDAC4 residues 1–747 (55.8±6.6, n =8) or HDAC4 residues 1–129 (61.4±6.8, n =6) was significantly greater, and HDAC4* exhibited by far the greatest efficiency in saving rd1 rods (105.5±12.9, n =6). HDAC4 N-terminal alleles exhibit greater protein stability To elucidate the differential protective effects evident in HDAC4 deletion alleles, we assayed HDAC4 protein levels using anti-HDAC4 immunohistochemistry at P12, when most rods still remain in rd1 mice. HDAC4 immunoreactivity for the N-terminal alleles was significantly higher than that observed for the full-length HDAC4 in the transfected areas labelled by co-electroporated CAG-GFP ( Fig. 2a ). Normalized HDAC4 immunoreactivity for the various HDAC4 N-terminal constructs ( Fig. 2b ), and elevated protein levels relative to the full-length HDAC4 ( Fig. 2c,d ) in electroporated retinas correlated positively with their efficiencies in saving rd1 rods. The expression of endogenous HDAC4 was not detected in rd1 retinas at P12 ( Fig. 2c and Discussion). The higher protein levels of HDAC4 N-terminal alleles were not due to differences in mRNA levels as measured by quantitative PCR ( Fig. 2e ). 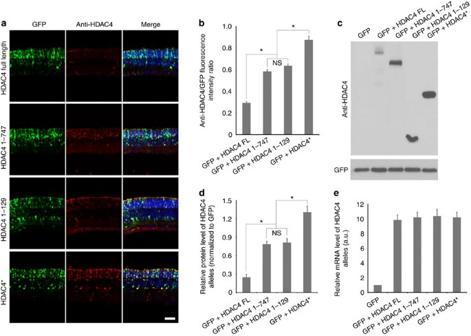Figure 2: Protein expression levels of HDAC4 Full Length and HDAC4 deletion alleles. (a) Assay of HDAC4 expression using anti-HDAC4 immunohistochemistry in the electroporated rd1 retinas at P12. Scale bar, 40 μm. (b) The intensity of anti-HDAC4 immunofluorescence was quantified as a ratio to the fluorescence intensity of co-expressed GFP. *P<0.01. Data are presented as mean±s.d.,n=3. (c) Assay of HDAC4 expression at P12 using anti-HDAC4 western blots in the electroporated rd1 retinas, and quantified (d) after normalization to the co-expressed GFP. *P<0.01. Data are presented as mean±s.d.,n=3. (e) Quantitative PCR analysis of mRNA levels of HDAC4 alleles at P12 in the electroporated rd1 retinas.n=3. Full scan images of western blot data are provided inSupplementary Fig. 10. Figure 2: Protein expression levels of HDAC4 Full Length and HDAC4 deletion alleles. ( a ) Assay of HDAC4 expression using anti-HDAC4 immunohistochemistry in the electroporated rd1 retinas at P12. Scale bar, 40 μm. ( b ) The intensity of anti-HDAC4 immunofluorescence was quantified as a ratio to the fluorescence intensity of co-expressed GFP. * P <0.01. Data are presented as mean±s.d., n =3. ( c ) Assay of HDAC4 expression at P12 using anti-HDAC4 western blots in the electroporated rd1 retinas, and quantified ( d ) after normalization to the co-expressed GFP. * P <0.01. Data are presented as mean±s.d., n =3. ( e ) Quantitative PCR analysis of mRNA levels of HDAC4 alleles at P12 in the electroporated rd1 retinas. n =3. Full scan images of western blot data are provided in Supplementary Fig. 10 . Full size image HDAC4 protein is unstable as it is subjected to caspase-dependent cleavage [25] , [26] , as well as polyubiquitination and proteasome degradation [27] . This raised the possibility that the greater protective effects observed for the HDAC4 N-terminal alleles might be due to their increased protein stability. To examine the stability of HDAC4 proteins, we expressed full-length HDAC4 or HDAC4 N-terminal alleles in transfected HEK293T cells and measured protein levels using western blots. The decay in protein was monitored over time following treatment with a protein synthesis inhibitor, cycloheximide, initiated at 20-h post transfection ( Fig. 3a,b ). Full-length HDAC4 protein was degraded fairly rapidly, as only ∼ 20% of the protein remained 6 h after cycloheximide treatment. The endogenous expression of HDAC4 was not detected in 293T cells transfected with GFP or empty vector controls ( Supplementary Fig. 3 ). By contrast, residues 1–129 and residues 1–747 of HDAC4 were more stable, with ∼ 75% of the protein detected under the same conditions. HDAC4* was the most stable allele with barely detectable protein degradation when protein synthesis was blocked during the 6 h time frame. The increased protein stability of the various HDAC4 alleles ( Fig. 3b ) correlated positively with their greater abundance after electroporation ( Fig. 2b,d ), and their ability to preserve rods from degeneration in rd1 mice ( Fig. 1d ). 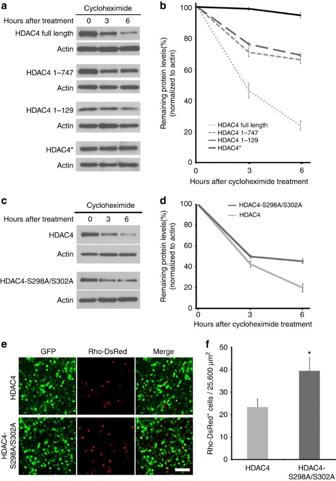Figure 3: Enhanced HDAC4 protein stability is correlated with greater rod protection efficiency. (a) Protein decay assay of HDAC4 Full Length and deletion alleles. HEK293T cells were transfected with CAG-HDAC4 or CAG-HDAC4 deletion constructs for 20 h before treatment with cycloheximide (100 μg ml−1) for 3 or 6 h. Cell lysates were immunoblotted for HDAC4. The same immunoblot membranes were stripped and re-probed for actin. (b) Protein levels were quantified by densitometry after normalization to actin. Data are presented as mean±s.d.,n=3. (c) Protein decay assay for HDAC4 and HDAC4-S298A/S302A mutant. HEK293T cells were transfected with CAG-HDAC4 or CAG-HDAC4-S298A/S302A for 20 h before treatment with cycloheximide (100 μg ml−1) for 3 or 6 h. Cell lysates were immunoblotted for HDAC4. The same immunoblot membranes were stripped and re-probed for actin. (d) Protein levels were quantified by densitometry after normalization to actin. Data are presented as mean±s.d.,n=3. (e) HDAC4-S298A/S302A saved more rd1 rods in comparison to the wild-type HDAC4 at P50. Scale bar, 40 μm. (f) Quantification of the preserved rods per 25,600 μm2on the flat-mount retina. *P<0.01. Data are presented as mean±s.d.,n=3. Full scan images of western blot data are provided inSupplementary Fig. 10. Figure 3: Enhanced HDAC4 protein stability is correlated with greater rod protection efficiency. ( a ) Protein decay assay of HDAC4 Full Length and deletion alleles. HEK293T cells were transfected with CAG-HDAC4 or CAG-HDAC4 deletion constructs for 20 h before treatment with cycloheximide (100 μg ml −1 ) for 3 or 6 h. Cell lysates were immunoblotted for HDAC4. The same immunoblot membranes were stripped and re-probed for actin. ( b ) Protein levels were quantified by densitometry after normalization to actin. Data are presented as mean±s.d., n =3. ( c ) Protein decay assay for HDAC4 and HDAC4-S298A/S302A mutant. HEK293T cells were transfected with CAG-HDAC4 or CAG-HDAC4-S298A/S302A for 20 h before treatment with cycloheximide (100 μg ml −1 ) for 3 or 6 h. Cell lysates were immunoblotted for HDAC4. The same immunoblot membranes were stripped and re-probed for actin. ( d ) Protein levels were quantified by densitometry after normalization to actin. Data are presented as mean±s.d., n =3. ( e ) HDAC4-S298A/S302A saved more rd1 rods in comparison to the wild-type HDAC4 at P50. Scale bar, 40 μm. ( f ) Quantification of the preserved rods per 25,600 μm 2 on the flat-mount retina. * P <0.01. Data are presented as mean±s.d., n =3. Full scan images of western blot data are provided in Supplementary Fig. 10 . Full size image Phosphorylation of HDAC4 at Ser 298 and Ser 302 promotes polyubiquitination and proteasome degradation. The HDAC4-S298A/S302A mutant has Ser 298 and Ser 302 mutated to Ala, which mimics the dephosphorylated state of the protein and is therefore more stable than wild-type HDAC4 (ref. 27 ). Indeed, HDAC4-S298A/S302A was more stable, as it decayed more slowly than the wild-type HDAC4 protein in the presence of cycloheximide ( Fig. 3c,d ). To directly test the role of HDAC4 protein stability on rod survival, we examined whether HDAC4-S298A/S302A might lead to increased rod protection using in vivo electroporation in rd1 retinas at P0. Quantification of rod survival at P50 showed significantly more rods in HDAC4-S298A/S30-treated retinas (39.4±5.9 rods per 25,600 μm 2 , mean±s.d., n =3) than with wild-type HDAC4 (24.5±3.4 rods per 25,600 μm 2 , mean±s.d., n =3; Fig. 3e,f ). These results suggest that increased HDAC4 protein stability contributes to greater rod protection, presumably due to persistently higher levels of functional HDAC4 protein. Requirement of conserved glutamine residues for rod protection Glutamine-rich sequences have been implicated primarily in pathological roles in neurodegeneration, causing polyglutamine toxicity in Huntington’s disease and the formation of amyloid fibrils in Alzheimer’s disease [28] , [29] . To elucidate the physiological role of the glutamine-rich region of HDAC4, we examined the rod protection efficacy of HDAC4 1–129 19QA and HDAC4 1–129 7QA alleles, which had either 19 glutamines or the 7 most conserved glutamines mutated to alanines ( Fig. 4a ). HDAC4 residues 1–129 preserved many rods in rd1 mice at P50 following in vivo electroporation at P0, while mutation of either all 19 or the 7 most conserved glutamines completely abolished the rod protection effect ( Fig. 4b,c ). The loss of rod protection in the glutamine to alanine mutants was not due to reduced protein levels, as they were detected at a level comparable to HDAC4 residues 1–129, measured by western blots in transfected HEK293T cells ( Fig. 4d ). Our results indicate that the conserved glutamine residues are essential for HDAC4-mediated rod protection in rd1 mice. CtBP (C-terminal Binding Protein), a synaptic protein expressed in rods [30] , binds to a conserved P-X-D-L-S/R motif located in the glutamine-rich region of HDAC4 [31] . However, a mutant (HDAC4 1–129 M4, Fig. 4a ), defective in CtBP binding [31] , preserved as many rd1 rods as HDAC4 residues 1–129 ( Fig. 4b,c ), suggesting that the rod protection effect of HDAC4 does not involve its interaction with CtBP. 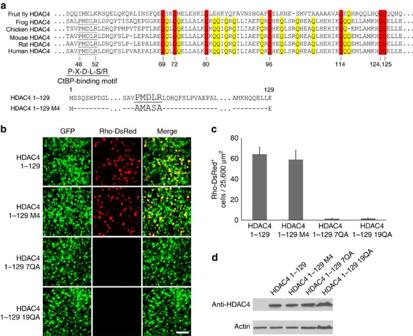Figure 4: The conserved glutamines in the HDAC4 N-terminal region are required for rod protection in rd1 mice. (a) Cross-species alignment of HDAC4 N-terminal protein sequences reveals conserved glutamine residues, which were mutated to alanines in HDAC4 1–129 19QA (mutated glutamines labelled in red and yellow) and 7QA (mutated glutamines labelled in red). CtBP-binding motif was also mutated in HDAC4 1–129 M4. (b) Rod protection by HDAC4 N-terminal mutants in comparison to its wild-type form in rd1 mice at P50. Scale bar, 40 μm. (c) Quantification of the preserved rods per 25,600 μm2on the flat-mount retina. Data are presented as mean±s.d.,n=6–10. (d) Expression of HDAC4 N-terminal mutants was detected by western blots in transfected HEK293T cells. Full scan images of western blot data are provided inSupplementary Fig. 10. Figure 4: The conserved glutamines in the HDAC4 N-terminal region are required for rod protection in rd1 mice. ( a ) Cross-species alignment of HDAC4 N-terminal protein sequences reveals conserved glutamine residues, which were mutated to alanines in HDAC4 1–129 19QA (mutated glutamines labelled in red and yellow) and 7QA (mutated glutamines labelled in red). CtBP-binding motif was also mutated in HDAC4 1–129 M4. ( b ) Rod protection by HDAC4 N-terminal mutants in comparison to its wild-type form in rd1 mice at P50. Scale bar, 40 μm. ( c ) Quantification of the preserved rods per 25,600 μm 2 on the flat-mount retina. Data are presented as mean±s.d., n =6–10. ( d ) Expression of HDAC4 N-terminal mutants was detected by western blots in transfected HEK293T cells. Full scan images of western blot data are provided in Supplementary Fig. 10 . Full size image HDAC5, another member of Class IIa HDACs, is highly homologous to HDAC4 in protein sequence and structure [32] . We tested the efficacy of HDAC5 residues 1–160, which contain a glutamine-rich region in its N-terminus, in saving rd1 rods by in vivo electroporation. Like HDAC4, many more rods were preserved by the short N-terminal region of HDAC5 ( Supplementary Fig. 4a,b ) in comparison to the full-length HDAC5. The rod protection effect mediated by HDAC4 or HDAC5 was not due to the overexpression of a random low-molecular-weight protein, as electroporation of Histone H3.1, a small protein of high stability expressed in the brain [33] , failed to preserve rd1 rods under the same conditions ( Supplementary Fig. 4a,b ). HDAC4 suppresses multiple photoreceptor death pathways Multiple pathways may be involved in photoreceptor death in rd1 mice, including disrupted calcium homoeostasis, excessive endoplasmic reticulum stress, increased reactive oxygen species, aberrant cell cycle progression, and overactivation of Calpain and Parp [34] , [35] , [36] , [37] . To investigate whether HDAC4 interacts with any of these pathways for rod protection, we used quantitative PCR to examine the mRNA expression profile of genes involved in photoreceptor death in rd1 mice at P12, when most photoreceptors remain. In comparison to GFP-electroporated rd1 retinas as a control, the expression of HDAC4*, the most effective form of HDAC4 in saving rd1 rods ( Fig. 1d ), did not significantly change the mRNA levels for photoreceptor-specific genes ( Fig. 5a ). We then categorized genes involved in photoreceptor death into three groups: transcription factors and cell cycle genes, genes involved in endoplasmic reticulum stress or oxidative stress, and cell death/apoptosis genes. Genes upregulated in rd1 retina relative to wild-type retina were indicated by a fold change of >1 (dashed lines in Fig. 5b–d ). 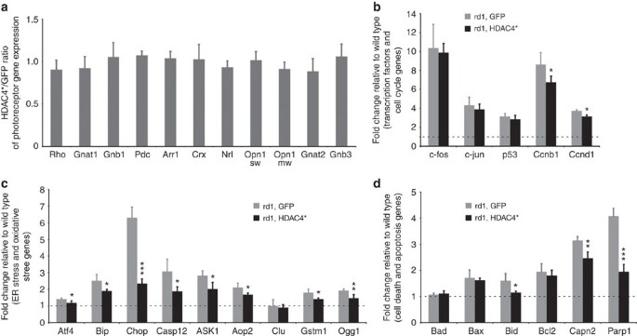Figure 5: Profiling gene expression in HDAC4*-electroporated rd1 retinas at P12 by quantitative PCR. (a) The mRNA levels of photoreceptor genes in HDAC4*-electroporated rd1 retinas relative to the GFP-electroporated rd1 retinas. (b) Assay of gene expression for transcriptional factors and cell cycle genes. (c) Assay of gene expression for endoplasmic reticulum stress and oxidative stress genes. (d) Assay of gene expression for cell death/apoptosis genes. Dashed lines inb–dindicate mRNA levels in the wild-type retina. *P<0.05, **P<0.01, ***P<0.001. Data are presented as mean±s.d.,n=3. Figure 5: Profiling gene expression in HDAC4*-electroporated rd1 retinas at P12 by quantitative PCR. ( a ) The mRNA levels of photoreceptor genes in HDAC4*-electroporated rd1 retinas relative to the GFP-electroporated rd1 retinas. ( b ) Assay of gene expression for transcriptional factors and cell cycle genes. ( c ) Assay of gene expression for endoplasmic reticulum stress and oxidative stress genes. ( d ) Assay of gene expression for cell death/apoptosis genes. Dashed lines in b – d indicate mRNA levels in the wild-type retina. * P <0.05, ** P <0.01, *** P <0.001. Data are presented as mean±s.d., n =3. Full size image Gene category 1: transcription factors and cell cycle genes ( Fig. 5b ). Transcription factors c-fos, c-jun and p53 are closely associated with retinal degeneration [38] , [39] . The mRNA levels for the three genes were strongly upregulated in the rd1 retina, however, HDAC4* had no effect on their expression in the rd1 retina. Cell cycle reactivation is a common feature of neuronal apoptosis during development and in neurodegenerative diseases [40] . Aberrant cell cycle progression was also proposed to be a cause of photoreceptor degeneration in rd1 mice [41] . Two cell cycle genes, Ccnb1 and Ccnd1 , were upregulated in the rd1 retina, and HDAC4* treatment significantly reduced the upregulation of both Ccnb1 and Ccnd1. Gene category 2: endoplasmic reticulum stress and oxidative stress genes ( Fig. 5c ). Activation of endoplasmic reticulum stress genes, including Atf4, Bip, Chop and Caspase-12, is implicated in degenerating photoreceptors in rd1 mice [42] . Similarly, genes involved in oxidative stress, including Aop2 , Gstm1 and Ogg1 , are also activated during photoreceptor degeneration [43] , [44] . Similarly, upregulation of ASK1 can be triggered by both endoplasmic reticulum stress and oxidative stress [45] . Consistent with previous findings, significant upregulation of this gene category was detected in the control GFP-treated rd1 mice. Noticeably, HDAC4* treatment attenuated the upregulation of these stress genes, especially the level of Chop expression. Gene category 3: cell death/apoptosis genes ( Fig. 5d ). The Bcl-2 family, which contains both pro-apoptotic ( Bad , Bax and Bid ) and anti-apoptotic ( Bcl2 ) genes, regulates the mitochondrial pathway of apoptosis by controlling the permeabilization of the outer mitochondrial membrane. The ratio of the two subsets determines the susceptibility of cells to cell death signals [46] . Significantly, the upregulation of the pro-apoptotic gene Bid was reduced by HDAC4* treatment. Calpain is a group of calcium-dependent cysteine proteases with substrates that include proteins regulating apoptosis such as PARP and AIF. Calpain is strongly activated in degenerating rd1 photoreceptors in rd1 mice [47] . PARP, poly (ADP-ribose) polymerase, an enzyme involved in DNA repair, is excessively activated in rd1 mice leading to caspase-independent cell death [48] , [49] . HDAC4* treatment attenuated the upregulation of both Calpain2 and Parp1. Our results indicate that HDAC4* treatment suppressed multiple cell death pathways involved in photoreceptor degeneration in rd1 mice. To determine whether the endogenous HDAC4 is required for HDAC4*-mediated rod survival in rd1 mice, we utilized a plasmid containing a short hairpin RNA to knockdown the expression of the native HDAC4 while co-electroporating an allele of HDAC4* resistant to the shRNA [11] . No significant reduction was seen in the number of preserved rd1 rods at P50 when endogenous HDAC4 expression was knocked down ( Supplementary Fig. 5 ). HDAC4 shuttles between the nucleus and cytoplasm [50] , [51] . It functions as a transcriptional repressor to regulate bone and muscle differentiation in the nucleus [17] , [18] , [52] , [53] . To investigate whether HDAC4 exerted its rod protection effect by engaging in activities in the nucleus or cytoplasm, we examined the localization of electroporated HDAC4 alleles in rd1 mice at P12 using fluorescence confocal microscopy. In addition to the cytoplasmic distribution, the co-electroporated GFP was also observed in the nucleus revealing the typical heterochromatin structure of rods. In comparison to the GFP localization, the full-length HDAC4 and HDAC4 N-terminal deletion alleles were mainly seen in the cytoplasm of the electroporated rods ( Supplementary Fig. 6 ). Our results indicate that HDAC4 functions in the cytoplasm to protect rd1 rods. HDAC4 acts in a cell-autonomous manner to protect rd1 rods Many non-photoreceptor cells, including bipolar cells, Müller glial cells and amacrine cells, are transfected by in vivo electroporation. To distinguish whether HDAC4 preserved rd1 rods through a cell-autonomous process or indirectly due to its expression in other cell types, we utilized a Cre-recombinase responsive expression system for cell-type-specific expression of HDAC4* ( Fig. 6a ) with a plasmid containing a ubiquitous CAG promoter and a floxed ‘stop cassette’. Rod-specific expression of HDAC4 was achieved by co-electroporation of Rho-Cre, a Cre-expression plasmid driven by the rhodopsin promoter [21] , [54] . Rods (83.2±10.7, n =3) were preserved in rd1 mice at P50 only in the presence of Rho-Cre ( Fig. 6b,c ). As the rhodopsin promoter becomes active when rod precursors differentiate to mature rods [54] , our results suggest that HDAC4 can be introduced at late postnatal stages to preserve rd1 rods in a cell-autonomous manner. 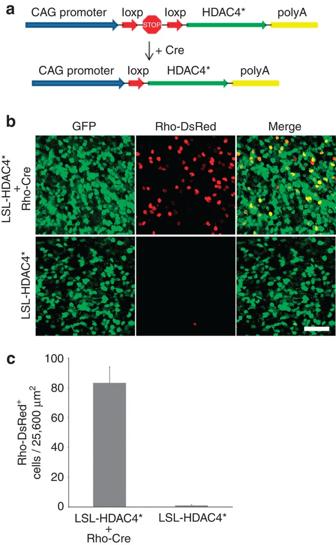Figure 6: HDAC4 acts cell-autonomously to protect rd1 rods. (a) Schematic illustration of a Cre-responsive expression system to restrict HDAC4 expression in rods. (b) Assay of rod survival at P50 in the presence and absence of Rho-Cre. Scale bar, 40 μm. (c) Quantification of rod survival per 25,600 μm2on the flat-mount retina. Data are presented as mean±s.d.,n=3. Figure 6: HDAC4 acts cell-autonomously to protect rd1 rods. ( a ) Schematic illustration of a Cre-responsive expression system to restrict HDAC4 expression in rods. ( b ) Assay of rod survival at P50 in the presence and absence of Rho-Cre. Scale bar, 40 μm. ( c ) Quantification of rod survival per 25,600 μm 2 on the flat-mount retina. Data are presented as mean±s.d., n =3. Full size image HDAC4* saves cone photoreceptors and restores visual function Electroporation in the neonatal mouse retina results in transfection of many rods, but few cones [21] . Rd1 rods preserved by HDAC4 are unlikely to function due to the mutation in the rod-specific gene PDE6β , which encodes a key enzyme in the rod phototransduction cascade. Rods mediate vision in dim light, whereas cones are responsible for daylight vision and visual acuity. RP patients maintain functional vision after rod degeneration for a long period of time due to the remaining function of cones, which are genetically normal. To investigate whether HDAC4 gene transfer saves cones as well as rods, and as a result, may restore visual function, we generated transgenic mice that express HDAC4* in FVB mice (a mouse strain homozygous for the rd1 mutation). HDAC4* expression was driven by a broadly active promoter, CAG, generating a photoreceptor-dominant expression pattern in a transgenic context [55] . An IRES (internal ribosome entry site) sequence was included in the transgenic construct ( Fig. 7a ) to simultaneously express GFP as a reporter for the HDAC4* transgene expression. We assayed transgene expression using western blots at P10, when most photoreceptors remain. While the endogenous HDAC4 was detected at a comparable expression level in HDAC4* transgenic mice and their non-transgenic littermates, HDAC4* and GFP were only detected in the HDAC4* transgenic mice, with HDAC4* expressed at a level about three times that of endogenous HDAC4 ( Fig. 7b ). We next examined transgene expression by anti-HDAC4 immunohistochemistry or GFP fluorescence in P10 retinal sections ( Fig. 7c ). HDAC4 immunoreactivity and GFP were detected predominantly in the perinuclear space of the outer nuclear layer of photoreceptors and the outer and inner segments of photoreceptors ( Fig. 7d ). Transgene expression, indicated by the GFP reporter, was evident in both rods labelled by anti-rhodopsin immunoreactivity ( Fig. 7e ), and cones labelled by anti-red/green cone opsin immunoreactivity ( Fig. 7f ). Transgene expression was also weakly detected in a subset of other cell types in the inner nuclear layer ( Supplementary Fig. 7 ). 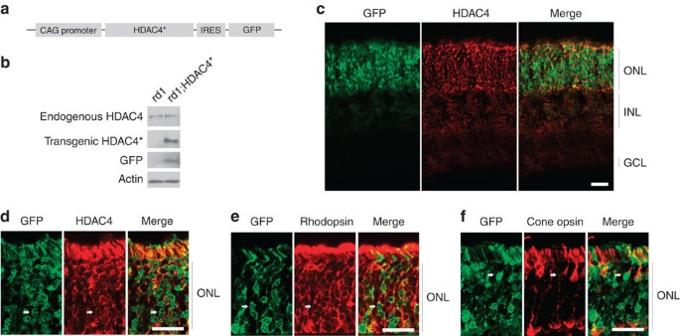Figure 7: Construction of HDAC4* transgenic mice. (a) Schematic representation of HDAC4* transgenic construct design. (b) Immunoblotting analysis of transgene expression in rd1;HDAC4* transgenic mice at P10. (c–f) Immunohistochemistry analysis of transgene expression in rd1;HDAC4* transgenic mice at P10 on retinal sections. Scale bar, 20 μm. (c,d) Detection of HDAC4 immunoreactivity and the GFP reporter. (e) Arrows: transgene expression in rods labelled by anti-rhodopsin immunohistochemistry. (f) Arrows: transgene expression in cones labelled by red/green cone opsin immunohistochemistry. Full scan images of western blot data are provided inSupplementary Fig. 10. Figure 7: Construction of HDAC4* transgenic mice. ( a ) Schematic representation of HDAC4* transgenic construct design. ( b ) Immunoblotting analysis of transgene expression in rd1;HDAC4* transgenic mice at P10. ( c – f ) Immunohistochemistry analysis of transgene expression in rd1;HDAC4* transgenic mice at P10 on retinal sections. Scale bar, 20 μm. ( c , d ) Detection of HDAC4 immunoreactivity and the GFP reporter. ( e ) Arrows: transgene expression in rods labelled by anti-rhodopsin immunohistochemistry. ( f ) Arrows: transgene expression in cones labelled by red/green cone opsin immunohistochemistry. Full scan images of western blot data are provided in Supplementary Fig. 10 . Full size image Photoreceptor degeneration starts in the centre and propagates to the periphery in rd1 mice [4] . We examined rod and cone photoreceptor survival at P42 in HDAC4* transgenic mice in comparison to their non-transgenic littermates by counting anti-rhodopsin immunoreactive cells or peanut agglutinin (a cone marker)-labelled cells in four retinal quadrants (dorsal, ventral, temporal and nasal) at two distances (700 and 1,400 μm) from the centre of the retina ( Supplementary Fig. 8 ). For rod survival at 700 μm from the centre of the retina ( Fig. 8a,b ), <10 rods remained in each of the four quadrants from non-transgenic littermates, while >100 rods were scored in corresponding areas in HDAC4* transgenic mice ( n =8). At 1,400 μm from the centre of the retina ( Fig. 8c,d ), 25–50 rods remained in the non-transgenic littermates compared with 180–250 scored rods in the HDAC4* transgenic mice ( n =8). For cone survival at 700 μm ( Fig. 9a,b ) or 1,400 μm ( Fig. 9c,d ) from the centre of the retina, HDAC4* expression significantly increased cone density in all four quadrants of the retina in HDAC4* transgenic mice compared with their non-transgenic littermates ( n =8). 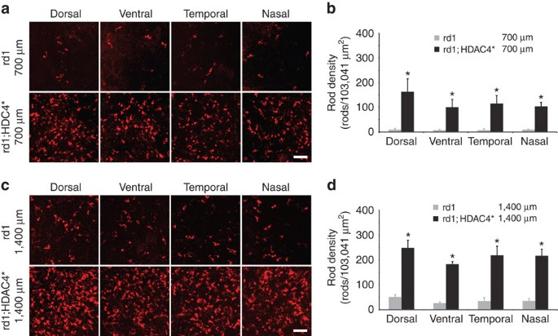Figure 8: Prolonged rod survival in HDAC4* transgenic mice. (a,c) Detection of rod photoreceptors in HDAC4* transgenic mice and their non-transgenic littermates at P42 by anti-rhodopsin immunohistochemistry on retinal flat mounts at 700 μm (a) or 1,400 μm (c) from the centre of the retina. Scale bar, 60 μm. (b,d) The number of rods was quantified in the four retinal quadrants (dorsal, ventral, temporal and nasal) at 700 μm (b) or 1,400 μm (d) from the centre of the retina. *P<0.01. Data are presented as mean±s.d.,n=8. Figure 8: Prolonged rod survival in HDAC4* transgenic mice. ( a , c ) Detection of rod photoreceptors in HDAC4* transgenic mice and their non-transgenic littermates at P42 by anti-rhodopsin immunohistochemistry on retinal flat mounts at 700 μm ( a ) or 1,400 μm ( c ) from the centre of the retina. Scale bar, 60 μm. ( b , d ) The number of rods was quantified in the four retinal quadrants (dorsal, ventral, temporal and nasal) at 700 μm ( b ) or 1,400 μm ( d ) from the centre of the retina. * P <0.01. Data are presented as mean±s.d., n =8. 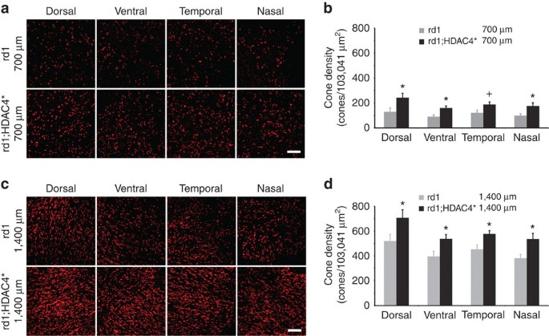Figure 9: Prolonged cone survival in HDAC4* transgenic mice. (a,c) Detection of cone photoreceptors in HDAC4* transgenic mice and their non-transgenic littermates at P42 by peanut agglutinin staining on retinal flat mounts at 700 μm (a) or 1,400 μm (c) from the centre of the retina. Scale bar, 60 μm. (b,d) The density of cones was quantified in the four retinal quadrants (dorsal, ventral, temporal and nasal) at 700 μm (b) or 1,400 μm (d) from the centre of the retina.+P<0.05; *P<0.01. Data are presented as mean±s.d.,n=8. Full size image Figure 9: Prolonged cone survival in HDAC4* transgenic mice. ( a , c ) Detection of cone photoreceptors in HDAC4* transgenic mice and their non-transgenic littermates at P42 by peanut agglutinin staining on retinal flat mounts at 700 μm ( a ) or 1,400 μm ( c ) from the centre of the retina. Scale bar, 60 μm. ( b , d ) The density of cones was quantified in the four retinal quadrants (dorsal, ventral, temporal and nasal) at 700 μm ( b ) or 1,400 μm ( d ) from the centre of the retina. + P <0.05; * P <0.01. Data are presented as mean±s.d., n =8. Full size image We examined whether HDAC4-mediated photoreceptor protection leads to improved visual function by recording electroretinograms (ERGs) in HDAC4* transgenic mice in comparison to their non-transgenic littermates in the same FVB strain background at P30. Scotopic ERG recordings were performed in dark-adapted animals with increasing light intensities from −3.6 to 2.9 log cd s m −2 . In wild-type mice, dim light flashes between −4.0 and −2.0 log cd s m −2 elicit responses from rods while cones start to be activated by brighter light stimuli [56] , [57] . Compared with typical ERG responses recorded from C57BL/6 wild-type mice ( Fig. 10a ), no ERG response was detected in either dim or higher light intensities from non-transgenic rd1 mice ( Fig. 10b ). In HDAC4* transgenic mice, no significant ERG response was elicited in lower light intensities until the light intensity increased to 1.4 log cd s m− 2 ( Fig. 10c,d ), indicating recovered function from cones. We further introduced the expression of a wild-type allele of PDE6β by in vivo electroporation in HDAC4* transgenic mice. The ERG recordings still showed no improved rod function in the PDE6β -electroporated HDAC4* transgenic mice ( Supplementary Fig. 9 ). The lack of recovery in rod function might be due to a limited number of PDE6β-transfected rods that appear in small patches typically generated by electroporation, resulting in undetectable responses by whole-field ERG recordings. We next recorded photopic ERGs to measure cone function in light-adapted animals. While photopic ERG responses were hardly detectable in the non-transgenic rd1 littermates, HDAC4* transgenic mice showed a noticeable photopic ERG response ( Fig. 10e ) with a significant b-wave amplitude (38.3±6.31 μV, n =11) ( Fig. 10f ). These results indicate that HDAC4* gene transfer in photoreceptors can partially restore cone-mediated visual function in rd1 mice. 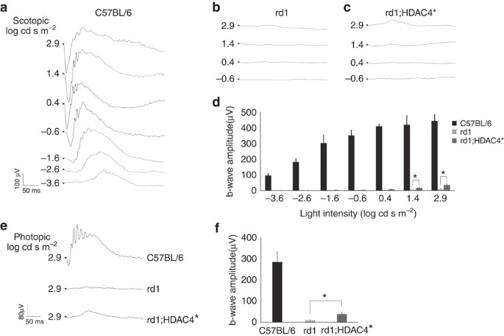Figure 10: Measurement of retinal function in HDAC4* transgenic mice. (a) Scotopic ERG was recorded at P30 in C57BL/6 wild-type retina, (b) non-transgenic rd1 retina and (c) rd1;HDAC4* transgenic retina. (d) Measured b-wave amplitudes of the scotopic ERG. (e) Photopic ERG was also recorded at P30 in C57BL/6 wild type, rd1;HDAC4* transgenic mice and their non-transgenic rd1 littermates. (f) Measured b-wave amplitudes of the photopic ERG. *P<0.01. Data are presented as mean±s.d.,n=5–11. Figure 10: Measurement of retinal function in HDAC4* transgenic mice. ( a ) Scotopic ERG was recorded at P30 in C57BL/6 wild-type retina, ( b ) non-transgenic rd1 retina and ( c ) rd1;HDAC4* transgenic retina. ( d ) Measured b-wave amplitudes of the scotopic ERG. ( e ) Photopic ERG was also recorded at P30 in C57BL/6 wild type, rd1;HDAC4* transgenic mice and their non-transgenic rd1 littermates. ( f ) Measured b-wave amplitudes of the photopic ERG. * P <0.01. Data are presented as mean±s.d., n =5–11. Full size image HDAC4 is a relatively large protein with many domains and a somewhat weak deacetylase domain [20] . It is shown to bind to several transcription factors and thereby play roles in muscle and bone development [17] , [18] , [52] , [58] . It also binds to Class I HDACs, such as HDAC1 and HDAC3 (refs 19 , 59 ). Here we show that none of these domains are required for the survival-promoting activity of HDAC4 in degenerating retinas. Surprisingly, a very short amino terminal domain with high glutamine content had as much rod protection function as the full-length HDAC4. In addition, an allele with some repeated elements from HDAC4, appended to the short glutamine-rich region, provided even greater protection. The basis of the differential rod protection effect is likely protein stability, which results in higher levels of HDAC4. Identification of the minimum functional domain of HDAC4 required for photoreceptor protection will likely aid in the design of a small protein therapeutic intervention for retinal degenerative diseases. HDAC4 is a dynamic protein with a regulated short half-life under normal conditions. The stability of HDAC4 is regulated by caspase-mediated cleavage at Asp-289 as the prime cleavage site [25] and polyubiquitination–proteasome degradation triggered by phosphorylation at Ser-298 and Ser-302 (ref. 27 ). We found that HDAC4 amino terminal alleles preserved more rods, and were more stable, than the HDAC4 full-length protein, establishing a positive correlation between protein stability and rod protection efficiency. The HDAC4-S298A/S302A mutant, which is resistant to ubiquitination–proteasome degradation and is thus more stable, also showed a greater effect in preserving rd1 rods relative to the wild-type allele. HDAC4*, the most stable form with high glutamine content, is the most efficient in saving rd1 rods. HDAC4 protein stability may contribute to greater efficiency in promoting photoreceptor survival, possibly due to higher protein levels. In rd1 mice, massive degeneration of rod photoreceptors starts around P10. Accumulation of cGMP, due to the rd1 mutation in PDE6β , is considered the trigger for rod death. While showing common features of apoptosis [60] , [61] , such as DNA fragmentation, the exact mechanism leading to photoreceptor degeneration remains elusive. Cytochrome c-mediated apoptotic pathway may not play a critical role as its release from mitochondria was not detected in the rd1 retina [62] . Multiple pathways may be implicated in the photoreceptor degeneration. Our results indicate that HDAC4 may interfere with at least several pathways by suppressing the expression of genes that are upregulated in degenerating photoreceptors. Interestingly, the endogenous expression of HDAC4 was significantly downregulated during photoreceptor degeneration in the rd1 retina as we detected it at P10 ( Fig. 7b ), but were unable to do so at P12 ( Fig. 2c ). The reduced expression of the endogenous HDAC4 in rd1 mice may have contributed to the fast cell death of rods as HDAC4 is required for the survival of rods and bipolar cells in normal retina [11] . Retinitis pigmentosa can lead to complete blindness, due to dysfunction and then death of both rod and cone photoreceptors, with no effective treatment currently available. Rd1 mice, which exhibit a pathology very similar to that of humans, provide an invaluable animal model for the evaluation of therapies for this disease. RP is genetically heterogeneous, with many of the disease mutations in rod-specific genes, including those essential for rod phototransduction, such as rhodopsin and PDE6β . Cones, genetically and functionally normal in many cases of RP, degenerate secondarily to rod death. Several hypotheses have been proposed to explain why normal cones die in RP, which include: the lack of rod-derived trophic factors [63] , the release of toxic factors by dying rods [64] , the compromised contact-mediated structure between the retina and the retinal pigmented epithelium [65] and poor nutritional support for cones [66] . Saving cones is key to preserving the vision of RP patients. Several approaches have prolonged the survival of cones in rd1 mice. These include treatments with calcium channel blockers [6] , antioxidants [7] and the manipulation of cell cycle regulators [41] , all of which have been shown to preserve cone function, as indicated by ERG measurements. We found that HDAC4* prolonged the survival of cones in transgenic mice harbouring the rd1 mutation. Significantly, HDAC4*-mediated cone photoreceptor protection generated a photopic ERG response. HDAC4* gene transfer thus may provide a potential treatment for photoreceptor disease by prolonging the survival of photoreceptors. Compared with the fast rod death in rd1 mice, cones are insensitive to light long before they die. Introduction of halorhodopsin, an optogenetic protein, into rd1 cones restored light sensitivity to cones, as well as vision [67] . The combination of HDAC4 and halorhodopsin might provide both greater survival as well as prolonged function in any disease where photoreceptors lose light responses and degenerate. Constructs and retinal electroporation HDAC4 and various HDAC4 deletion alleles were constructed into the pCAGEN vector (Addgene) for in vivo electroporation. In short, newborn rd1 mouse pups (FVB strain) were anaesthetised by chilling on ice, and a small incision was made in the eyelid with a 30-gauge needle to expose the eyeball. DNA mix (1 μg μl −1 of each plasmid) was injected into the subretinal space with a Hamilton syringe followed by electroporation with a tweezer-type electrode and the ECM830 (BTX) pulse generator applying five 80 V square pulses for 50 ms duration each pulse and 950 ms intervals. Immunoprecipitation and immunoblotting from transfected cells HEK293T cells (ATCC) were cultured in DMEM (Gibco) with 10% FBS (Sigma) and penicillin-streptomycin (Lonza). Transfection was performed using Lipofectamine 2000 (Life Technologies). For immunopurification, CAG-HDAC4* transfected cells were collected 48-h post transfection. Cleared cell lysates were incubated with an anti-HDAC4 antibody raised against residues 1–19 of human HDAC4 (Sigma), and bound proteins were precipitated with Protein A/G plus agarose beads (Santa Cruz Biotechnology). For immunoblotting, retinal tissues or cells were lysed by boiling in 2% SDS Sample Buffer. Proteins were separated by SDS–polyacrylamide gel electrophoresis and electro-transferred onto PVDF (polyvinylidene difluoride) membranes (Bio-Rad). Primary antibody: HDAC4 (Sigma, 1/2,000), GFP (Thermo scientific, 1/2,000), β-Actin (Thermo Scientific, 1/3,000). Secondary antibody: HRP-linked anti-mouse IgG (Cell Signaling, 1/4,000). The antigens were detected using Pierce ECL Western Blotting Substrate (Thermo Scientific) and HyBlot CL autoradiography film (Denvilles Scientific). Full scan images of western blots data are provided in Supplementary Fig. 10 . Mass spectrometry In gel protein digestion: the SDS–polyacrylamide gel electrophoresis-separated protein band of HDAC4* was excised and washed with acetonitrile/ammonium bicarbonate/acetonitrile buffers. After washing, the gel was speedvaced to dryness, rehydrated with 45 μl of 0.0067 μg trypsin (Promega), and digested at 37 °C for 16 h. Liquid chromatography–mass spectrometry (LC–MS/MS) on the LTQ Orbitrap: LC–MS/MS analysis was performed on a Thermo Scientific LTQ Orbitrap equipped with a Waters nanoAcquity UPLC system. Sample trapping was done at 15 μl min −1 , 99% Buffer A (100% water and 0.1% formic acid) for 1 min on a Waters Symmetry C18 180 μm × 20 mm trap column. Peptide separation was at 300 nl min −1 on a1.7 μm, BEH130 C18, 75 μm × 250 mm nanoAcquity UPLC column (35 °C). A linear gradient was run at initial conditions. MS was acquired in the Orbitrap using 1 microscan, 30,000 resolution and a maximum inject time of 900 followed by six data dependant MS/MS acquisitions in the ion trap. The data was searched using Mascot Distiller and the Mascot search algorithm. Immunohistochemistry and fluorescence microscopy Retinas were fixed in 4% paraformaldehyde in PBS for at least 30 min at room temperature for retinal flat mount or cryosection. Primary antibodies: HDAC4 (Sigma, 1:200), Rhodopsin (Rho4D2, 1:100), Red/Green opsin (Millipore, 1:200) and biotin-conjugated Peanut agglutinin (1:300). Secondary antibodies: DyLight 594/647-conjugated affiniPure antibodies or streptavidin (Jackson ImmunoResearch). Confocal images were acquired using a Zeiss LSM 510 EXCITER microscope. Images were analysed in Image J. RNA extraction and quantitative PCR Total RNAs from electroporated retinas were isolated using TRIzol reagent (Life Technologies) according to manufacturer’s instructions. cDNAs were synthesized with the RETROscript kit (Life Technologies) kit and then used as templates for PCR amplification. Real-time PCR was performed using SsoFas EvaGreen supermix (Bio-Rad) reagent with iCycler iQ Real-Time PCR Detection System. Primer sequences are listed in Supplementary Table 1 . Generation of HDAC4* transgenic mice and genotyping All animal experiments were performed in accordance with the animal protocol approved by the Institutional Animal Care and Use Committee of Yale University. Linearized HDAC4* pCAGIG vector (Addgene) was used for FVB mouse zygote pronuclear microinjection (Gene Targeting and Transgenic Facility, University of Connecticut Health Center). Transgenic founders were identified by genotyping with PCR primers: AAACACGATGATAATATGGC and TCATGTGGTCGGGGTAG. Established HDAC4* transgenic lines are maintained by breeding hemizygous males to non-transgenic FVB females. Male and female C57BL/6 mice at 8–10 weeks of age were purchased from The Jackson Laboratory (Bar Harbor, Maine). ERG recordings ERGs were recorded using an UTAS visual electrodiagnostic system equipped with BigShot Ganzfeld stimulator (LKC Technologies). Mice were anaesthetised with a mix of ketamine (100 mg kg −1 ) and xylazine (10 mg kg −1 ) by intraperitoneal injection. Pupils were dilated with 1% tropicamide (Alcon) and 1% Atropine. A pair of platinum electrodes was placed on each cornea, a reference electrode was placed subcutaneously in the anterior scalp between the eyes, and a ground electrode was inserted into the tail. Corneal hydration was maintained by application of Blink Gel Tears lubricating eye drops (Abbott). For scotopic ERG, mice were dark-adapted and stimulated with flashes of increasing light intensity (−3.6, −2.6, −1.6, −0.6, 0.4, 1.4 and 2.9 log cd s m −2 ). For photopic ERG, mice were light-adapted for 15 min and stimulated with flashes (2.9 log cd s m −2 ) in the presence of a white background light (30 cd m −2 ). Signals were band-pass filtered between 0.3 and 100 Hz and averaged response from 16 single flashes were recorded and analysed. Statistical analysis Data are presented as mean±s.d. A two-tailed Student’s t -test was used to determine the statistical significance between different experimental groups. How to cite this article: Guo, X. et al. A short N-terminal domain of HDAC4 preserves photoreceptors and restores visual function in retinitis pigmentosa. Nat. Commun. 6:8005 doi: 10.1038/ncomms9005 (2015).